Nickel-catalyzed divergent Mizoroki–Heck reaction of 1,3-dienes Developing efficient strategies to realize divergent arylation of dienes has been a long-standing synthetic challenge. Herein, a nickel catalyzed divergent Mizoroki–Heck reaction of 1,3-dienes has been demonstrated through the regulation of ligands and additives. In the presence of Mn/NEt 3 , the Mizoroki–Heck reaction of dienes delivers linear products under Ni(dppe)Cl 2 catalysis in high regio- and stereoselectivities. With the help of catalytic amount of organoboron and NaF, the use of bulky ligand IPr diverts the selectivity from linear products to branched products. Highly aryl-substituted compounds can be transformed from dispersive Mizoroki–Heck products programmatically. Preliminary experimental studies are carried out to elucidate the role of additives. The transformation of metal aryl species is one of the most important topics in modern organometallics [1] , [2] , [3] , [4] . Taking advantage of the diversity from metal aryl species, a variety of valuable name reactions have been discovered to accomplish different arylations [5] , [6] , [7] , [8] . Among them, Mizoroki–Heck reaction has been recognized as an elegant strategy for carboarylations of alkenes [9] , [10] , [11] , [12] , [13] . However, most of current Mizoroki–Heck reactions focused on the arylation of mono alkenes [14] , [15] , [16] , [17] , [18] , [19] , [20] , [21] , [22] or using noble palladium catalysts [23] (Fig. 1a ). Therefore, it is of great interest to develop divergent arylations of more challenging molecules under earth abundant metal catalysts. Fig. 1: Transition metal-catalyzed arylations of 1,3-dienes. a Dehydroarylations of alkenes under transition metal catalysis. b Our previous work: Selective arylations of 1,3-dienes via Ni/Cr catalysis. c This work: Ni-catalyzed divergent Heck reactions of 1,3-dienes. Full size image As extensive feedstocks in nature and industry, the catalytic functionalization of 1,3-dienes is a straightforward strategy to build up the molecular complexity [24] , [25] , [26] , [27] , [28] , [29] , [30] , [31] , [32] , [33] , [34] , [35] , [36] , [37] . However, compared with that of mono alkenes, the arylation of dienes brings extra challenges in selective control owing to the existence of an additional C = C bond [38] , [39] , [40] . Theoretically, tremendous arylation products (Heck, hydroarylation [41] , [42] , [43] , [44] , [45] , [46] , and diarylation [47] , [48] , [49] , [50] , [51] , [52] , [53] , [54] , [55] , [56] , [57] , [58] products) with different regio- and stereo-isomers would be expected to be observed through the coupling of aryl halides and dienes. Under Ni/Cr cocatalysis, we previously developed selective diarylation of 1,3-dienes. Besides the desired diarylation product, minor Heck or hydroarylation products were also observed (Fig. 1b ) [59] . Similar side-products have also been observed by Koh et al. in their recent work on diarylation of aliphatic 1,3-dienes [60] . Inspired by these precedents [40] , [41] , [42] , [43] , [44] , [45] , [46] , [47] , [48] , [49] , [50] , [51] , [52] , [53] , [54] , [55] , [56] , [57] , [58] , [59] , we envisioned whether it would be possible to divert the reactivity of Ni−Ar species from diarylation to Heck reaction of dienes. Given the four reactive sites of 1,3-dienes, it will also be possible to obtain divergent regioisomers on Heck reaction. Here, we develop a divergent Heck reaction of 1,3-dienes under nickel catalysis (Fig. 1c ). Programmable transformations from dispersive Heck products have been demonstrated to construct a series of highly aryl-substituted compounds. 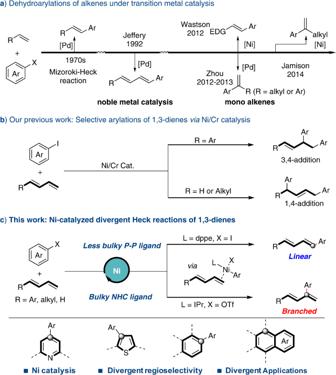Fig. 1: Transition metal-catalyzed arylations of 1,3-dienes. aDehydroarylations of alkenes under transition metal catalysis.bOur previous work: Selective arylations of 1,3-dienes via Ni/Cr catalysis.cThis work: Ni-catalyzed divergent Heck reactions of 1,3-dienes. Reaction optimization Aryl triflate 1a and diene 4a were chosen as model substrates for the investigation of divergent Heck reactions under nickel catalysis (Table 1 ). In the presence of Mn, a small amount of linear Heck product 5a (9% yield) was detected using Ni(dppe)Cl 2 as catalyst precursor accompanied by trace of branched Heck product 6a (1% yield) and hydroarylated products 7 – 9 (5% yield, entry 1). With the addition of NEt 3 , the yield of product 5a was increased from 9 to 15% (entry 2). Obvious impact on reactivity and selectivity was observed through the evaluation of other leaving groups (entries 3 and 4). When 4-methoxyphenyl triflate 1a was replaced by 4-iodoanisole 3a , 40% yield of 5a was obtained with excellent selectivity (entries 2 vs 4). As the amount of NEt 3 increased (MeCN/NEt 3 = 9:1), the yield of 5a could be improved to 63% in the presence of less manganese powder (entry 5). Given their ability in promoting the circulation of Ni catalyst, some inorganic salts were added to facilitate the reaction (entries 6 and 7) [61] . In terms of reactivity, NaCl emerged as the preferred additive for the formation of 5a (81% yield). Control experiments further confirmed that nickel was indispensable for this reaction (entry 8). Without the Mn powder, the yield of 5a decreased significantly (entry 9). Table 1 Optimization of reaction conditions. a Full size table When the reaction was conducted with Ni(0) precursor, it exhibited the similar results with that in the presence of Ni(II)/Mn combo (entry 10 vs 1). Replacing NEt 3 with Cs 2 CO 3 as base slightly increased the yield of 6a and inhibited the formation of linear product 5a (entry 11). With the aid of ligand IPr, milder condition (40 °C) and higher yield (31%) was achieved in the presence of catalytic amount of (Bpin) 2 (entries 12 and 13). Then, through the screening of various solvents and bases, 1,4-dioxane as solvent brought poor selectivities of 5a and 6a . But there was not much difference between DMF and MeCN (entries 13–15). When Cs 2 CO 3 was replaced by KOEt or LiOMe, undesirable hydroarylation and diarylation products increased distinctly (entries 16 and 17). Notably, the addition of catalytic amount of KO t Bu could further promote the reaction (46% yield of 6a ) (entry 18). Arylboron ( B1 ) showed more effective when compared these results with other organoboron agents (entry 19 and see SI for details). A combination of B1 and NaF led to an increase in the yield of 6a (74% yield) in DMF/Hexane (3:2 v/v ) (entry 20). Substrate scope With the optimized conditions in hand, we subsequently explored the scope of substrates in this divergent approach (Fig. 2 ). For linear Heck reaction, the 1,3-dienes bearing electron-donating groups on the aromatic ring, including Me ( 5b, 5h-5j ), Et ( 5c ), t Bu ( 5d ), NMe 2 ( 5 g ), all reacted with 4-iodoanisole smoothly and delivered the corresponding products in moderate to good yields with excellent selectivities. In comparison, electron-deficient substrates showed slightly low stereoselectivities ( 5e and 5f ). Notably, naphthyl and furyl substituted 1,3-dienes were also compatible with this transformation, leading to 1,4-diaryldienes in 70 and 72% yields, respectively. In addition, when using aliphatic 1,3-dienes ( E/Z = 1/1) for the coupling with 4-iodoanisole, product 5m could be successfully afforded in 66% yield and 9:1 stereoselectivity. Satisfyingly, the reaction also proceeded with naked 1,3-butadiene, which may provide an alternative route for the synthesis of 1-arylbutadienes and avoid the huge waste during traditional Wittig reactions. Not only the mono-substituted dienes, but also the 5o could be obtained from 1,2-disubstituted diene with high yield and selectivity under the standard condition. Lower reactivities and selectivities were obtained for isoprene and 1,3-disubstituted diene ( 5p and 5q ). Fig. 2: Substrate scope towards divergent Heck reactions. a Substrate scopes of dienes for linear products. b Substrate scopes of Ar-I for linear products. c Substrate scopes of dienes for branched products. d Substrate scopes of Ar-OTf for branched products. e Cascade Heck reactions. Isolated yields were given in all cases. Selectivities were >20:1 except for some cases with footnotes, which were determined by GC-FID or 1 H NMR analysis. a iodobenzene (9.0 mmol), 4a (6.0 mmol); b 3a (0.20 mmol), 1,3-diene (0.60 mmol); c Isolated yield of two steps (coversion of -CO 2 H to -CO 2 Me); d 1 (0.20 mmol), 4 (0.25 mmol), 4-CNC 6 H 4 Bneop ( B2 , 20 mol%) was used instead of B1 ; e A mixture of Z - and E -isomers of diene 4 was used; f 1 (0.25 mmol); g 1 (0.20 mmol), 4 (0.25 mmol), KO t Bu was used instead of NaF; h 1 (0.10 mmol), 4 (0.25 mmol), Ni(cod) 2 (20 mol%), IPr∙HCl (24 mol%), Cs 2 CO 3 (3.0 equiv. ), B1 (40 mol%), KO t Bu (40 mol%); i 3a (1.0 mmol), 1,3-butadiene (3.0 mmol), MeCN/NEt 3 (5.0 mL/0.60 mL = 9:1); j Ar-I (0.60 mmol), 5n (0.40 mmol), MeCN/NEt 3 (1.0 mL/0.11 mL = 9:1). Full size image Then the iodoarene substrates were explored (Fig. 2b ). A variety of iodoarenes bearing electron-withdrawing and electron-donating groups all underwent the desired cross-coupling smoothly. Generally, the corresponding linear Heck products were obtained with good to excellent yields, high stereoselectivities and exquisite regioselectivities ( 5r − 5 y and 5aa − 5hh , 60−92% yields). However, the coupling of methyl 4-iodobenzoate with 1,3-diene displayed moderate stereoselectivity ( 5z / 5z′ = 84/16). It should be noted that the bromo group, which could offer useful handles for further synthetic manipulations, was well compatible under the current conditions ( 5w ). Additionally, substrates bearing sensitive groups, such as carboxylic acid, aldehyde, unprotected indole and pyridines ( 5aa , 5ee , and 5ff-5hh ), were all applicable, highlighting the general tolerance of this nickel catalysis. To illustrate the practical utility of this strategy, a scale-up experiment under the standard conditions was performed to afford the corresponding product 5s in 1.05 g with 85% yield. Next, we sought out to assess the substrate scope towards branched arylation. In order to facilitate the separation of products and additives, 4-cyanophenylboron B2 was used instead of B1 in some cases. As illustrated in Fig. 2c , dienes with either electron-donating or electron-withdrawing substituents at the 4-position of phenyl ring all reacted with diene 4a in good reactivities and excellent regio- and stereo-selectivities ( 6a − 6f , 59–81% yields). In addition, 1,3-diene possessing ester group was well tolerated in this case, but minor hydroarylation product could be observed ( 6g/6g″ = 92:8). Similar to linear Heck reactions, aliphatic-1,3-dienes was also well applicable to this strategy ( 6h and 6i ). Depending on the E/Z ratio of diene substrates, the stereoselectivities of aliphatic products would be maintained. Although the less impressive result ( 6j ) was obtained for 1,4-disubstituted diene, 1,1′-diaryl-1,3-dienes showed good reactivities and regioselectivities for the current transformations and were not affected by steric hindrance of another aromatic ring (83% yield for 6k and 86% yield for 6l ). Meanwhile, the scope of aryl triflates in coupling with dienes was investigated under the Ni/IPr catalysis (Fig. 2d ). Generally, the reaction exhibited no obvious loss in both reactivities and selectivities when electron-rich or electron-deficient were subjected ( 6 m , 6n, 6o and 6t-6v ). Good yields and selectivities could also be achieved even when ortho-substituted aryl triflates were employed, regardless of their steric hindrance ( 6n and 6o ). In addition, substrates derived from estrone and diethylstilbestrol could also react smoothly to obtain corresponding branched products ( 6w and 6x ). Consecutive Heck reaction could even proceed from common material to deliver a hybrid of linear and branched diene (Fig. 2e ). Under condition A, linear diene 5n could be synthesized from 4-Iodoanisole and 1,3-butadiene with 36% yield in 1 mmol scale. Using bifunctional coupling reagent 4-iodophenyl triflate, nickel catalysis could selectively cleave C−I bond rather than C−O bond in condition A to yield ( E,E )−1,4-diarydiene 5ii . Without the influence of the two C=C bonds of 5ii , polyene 6 y bearing linear and branched diene motifs was constructed in 71% yield under condition B. Transformations To demonstrate the synthetic utility of the diarylation products, concise syntheses of highly aryl-substituted compounds were performed from linear and branched dienes 5 and 6 (Fig. 3a ). Through a Ni-catalyzed dehydrogenative [4 + 2] cycloaddition between nitrile and branched arylated product 6 m , diaryl- and triaryl pyridines ( 11a and 11b ) could be accessed with 42 and 56% yields respectively [62] . Multisubstituted benzenes ( 12a and 12b ) were easily synthesized from 5 s and 6 m in 92 and 74% yields via Diels-Alder reaction and oxidation in one pot [63] . Meanwhile, diaryl thiophenes ( 13a and 13b ), which were potential pesticides, could also be accessed by an oxidative cyclization from inorganic sulfurating reagents K 2 S and diene 5a or 6a . Under nickel catalysis [64] , the hydroarylations of linear diene 5 s smoothly delivered diarylated products 14a and 14b which could be further converted to polyaryl thiophene 15 and naphthalene 16 [64] , [65] . Fig. 3: Divergent and programmable synthetic transformations of dienes. a Divergent constructions of highly aryl-substituted compounds. b Programmable constructions of poly (hetero)aromatic compounds. Full size image On the other hand, the linear poly (hetero)aromatic compounds, as important components of quasi-one-dimensional conducting polymers [66] , could be constructed programmatically from simple starting materials. The chemoselective coupling of bifunctional reagent 4-iodophenyl triflate with 1-phenyl-1,3-diene yielded the desired aryl triflate 17 . Subsequent Suzuki reactions of 17 with different (hetero)arylboronic acid gave ploy (hetero)aryl dienes 18 and 19 [67] . Through oxidative cyclizations, linear poly (hetero)aromatic compounds 20 and 21 were finally obtained in 96 and 64% yields (Fig. 3b ) [63] , [64] . Mechanistic investigations Corresponding control studies were carried out to shed light on the mechanistic insights. The chemoselectivities and regioselectivities of Ni catalysis on two leaving groups (I or OTf) were investigated under standard conditions A and B. Although good yield of 5a was obtained for PMP-I 3a in condition A, no expected product 5a or 6a was observed under condition B (Fig. 4a , entries 1 and 2). For aryl triflate 1a , less Heck product 5a was found in condition A than that of PMP-I 3a (entries 3 vs 1). Moreover, branched product 6a became the only product instead of 5a in condition B (entries 4 vs 3). These control experiments suggest that, the reactivity of linear arylation is positively correlated with the leaving ability of substituted group (I and OTf). While for branched Heck reaction, this reaction is chemospecific to the leaving group. In addition, regioselectivity is regulated by ligand or additives other than leaving groups. Fig. 4: Mechanistic studies of Heck reactions. a Control experiments. b Stereoconvergent Heck reactions of dienes. c The effect of ligands. d The capture and catalytic performance of Ni(0) species. e 31 P NMR spectra of control experiments. f The role of [Ar-B] species. g 19 F NMR spectra of control experiments. Full size image When submitting a Z / E mixture of diene isomers ( 4a/4a ′ = 1/1 and 4b/4b ′ = 1/2) to the Heck reaction conditions, only E products 5a and 6a were deserved and the yields were similar to that of results using ( E )-substrates (Fig. 4b ). Through the analysis of the recovered starting materials, the E/Z ratio of diene 4a did not change significantly under condition A, but only ( E )-diene 4b was recovered in 5% yield. In the absence of triflate 1a , only ( E) - 4b was recovered under condition B. The strong stereoconvergent effect implies that an interconversion between η 1 -allyl nickel and η 3 -allyl nickel species might be involved in the catalytic cycle of linear Heck reaction. And it indicates a fast isomerization from cis - to trans -diene 4 could occur in branched Heck reaction. From the evaluation of NHC ligands (Fig. 4c ), the less bulky ligand IMes displayed lower regioselectivity and reactivity ( L2 vs L1 ). But as the steric hindrance increases on one side of the ligand, the selectivity and yield would be slightly promoted ( L3 vs L2 ). When L1 was replaced by L4 which shows the only difference in donor properties, the yield of 6a decreased a little bit but the selectivity could still be maintained. It indicated that the steric hindrance of ligand has a more significant effect on the regioselectivity than electronic effect. There was no obvious reaction with the addition of L5 or L6 and it seems that the skeleton of ligand has a decisive influence on the reactivity. These conclusions have been supported by previous theoretical study [68] . Possibly due to energy difference of insertion transition states [69] , the use of phosphine ligands and bulky NHC ligands displayed the opposite selectivities. Next, further studies have been performed to capture possible intermediates and verify the effects of additives in this divergent Heck reaction. For linear Heck reaction of diene, treating stoichiometric Ni II (dppe)Cl 2 with Mn powder in MeCN/NEt 3 successfully provided Ni 0 (dppe) 2 which structure was confirmed through X-ray analysis (Fig. 4d ). With the aid of this prepared Ni 0 precursor Ni(dppe) 2 , the Heck reaction coupling between 3a and 4a could also proceed smoothly to deliver product 5a in 45% yield. Based on these observations, the linear Heck reaction might be initiated by the formation Ni(0) species in situ. Meanwhile, NEt 3 has shown important effect on enhancing the reactivity of current Ni-catalyzed linear Heck reaction (Table 1 ). Thus, 31 P NMR spectra of control experiments were then performed to probe the role of NEt 3 . As depicted in Fig. 4e , the chemical shift of Ni(dppe)Cl 2 in MeCN was found at 59.44 ppm. No new signal or chemical shift was found after the addition of Mn to the Ni(dppe)Cl 2 solution, indicating the difficulty of the Ni(II) precursor to be reduced to Ni(0) species by Mn powder alone in this case. However, a new peak at 43.87 ppm, which should be assigned to Ni 0 (dppe) 2 complex, could be successfully detected when NEt 3 was loaded. Therefore, this unexpected reduction indicates that NEt 3 not only served as a base in this transformation, but also may facilitate reduction process of Ni II precursor to Ni(0) species. For branched Heck reaction, organoboron also plays a crucial role on reactivity. Diboron compounds have been previously suggested to reduce Ni II to Ni 0 [51] , [54] . Using Ni(OTf) 2 instead of Ni(cod) 2 as catalyst precursor, aryl boron ( B1 ) did not show the same positive effect as diboron (B 2 neop 2 ) (Fig. 4f , entries 1 vs 2). It suggests that Ni II could not be reduced effectively by aryl boron. In the absence of organoboron additive, chelated solvent dimethoxy methane (DMM) favored the formation of 6a than DMF and MeCN (Fig. 4f , entries 3–5). Given the structural similarity between boron ester and DMM, it indicates that boron ester probably promote reaction through chelation on Ni catalyst. To figure out the role of aryl group on additive B1 , nonreductive i PrOB(OMe) 2 was used instead of B1 for branched dehydroarylation. The desired reaction occurred in the presence of the catalytic amount of NaF or KO t Bu and the latter gave a higher yield (Fig. 4f , entries 6–8) [70] . These results indicate that ionic ployalkoxyborate better promotes the branched Heck reaction than neutral organoborate. It also rules out the reductant role of arylboron B1 for Ni catalyst. Meanwhile, 19 F NMR studies of control experiments were performed to further confirm the chelation effect of borate (Fig. 4g ). The addition of Ni(OTf) 2 to B1 in DMF led a clear change from −110.67 ppm to −109.76 ppm in 19 F NMR spectra (Fig. 4g , I vs III). This downfield shift probably resulted from a decrease of electron density on fluorine atom of B1 . However, there was no obvious change on chemical shift of 19 F NMR signal by mixing Ni(cod) 2 with B1 in DMF. It suggests anionic organoborate preferentially coordinate with cationic Ni II species rather than neutral Ni 0 complex in the catalytic cycle. On the basis of the above observations, a plausible mechanism for the divergent arylation via nickel catalysis was proposed (Fig. 5 ). For linear Heck reaction, catalyst precursor Ni(dppe)Cl 2 is reduced to give active Ni(0) species A in situ by Mn powder and NEt 3 . Subsequently, an oxidative addition of iodoarene 3 with A yields aryl-Ni(II) complex B . Then, migratory insertion between complex B and 1,3-diene 4 gives allyl-nickel complex C or its ƞ 3 coordinated form E . Next, final β -H elimination from complex C affords linear Heck product 5 and Ni II species D . With the aid of Mn and NEt 3 , Ni 0 catalyst A is regenerated from Ni II species D to complete the catalytic cycle. Fig. 5: Proposed mechanism for divergent arylation via nickel catalysis. Through the regulation of dppe ligand, linear Heck product 5 is obtained in presence of Mn and NEt 3 . With the aid of bulky ligand IPr, the selectivity of reaction is switched to branched product 6 in presence of alkoxyborate. Full size image For branched Heck reaction promoted by IPr ligand (Fig. 5 , right), cationic Ni(II) species B′ is initially obtained from an oxidative addition of aryl triflate 1 with A . Meanwhile, the reaction of organoboron with base (NaF or KO t Bu) produces alkoxyborate E . Then a chelation of cationic Ni II species B ′ with anionic organoborate E ′ forms Ni(II) complex F′ . A subsequent migratory insertion of diene 4 into Ni-Ar F ′ yields an alkyl-nickel (II) species C′ . The steric hindrance between bulky ligand IPr and allylic motif impedes the formation of isomer C . Afterwards, product 6 and Ni II species D′ can be obtained through β -H elimination from complex C′ . With the help of Cs 2 CO 3 , a final reductive elimination from allyl-Ni III species D′ regenerates the Ni 0 catalyst A and alkoxyborate E′ for next catalytic cycle. It will be more challenging to realize the 1- and 2-arylation of dienes which probably requires special substrate or catalyst design. In this work, a divergent Heck reaction of 1,3-dienes with Ar-X (X = I or OTf) is developed under Ni catalysis. Through the regulation of dppe ligand, linear Heck products are successfully obtained in presence Mn and NEt 3 . The selectivity of reaction is efficiently switched to branched products by the combination of Ni(cod) 2 /IPr and alkoxyborate. A series of highly aryl-substituted compounds are constructed programmatically and concisely from our protocol. Besides, preliminary mechanistic studies provide clues for possible catalytic pathways and the role of additives. Further studies and application on this divergent arylation of dienes are underway in our laboratory. General procedure for Ni-catalyzed linear Heck reaction of 1,3-dienes In a glove box, a sealed tube was charged with iodoarene 3 (0.40 mmol), Ni(dppe)Cl 2 (0.02 mmol, 10 mol%), Mn (0.20 mmol, 1.0 equiv. ), NaCl (0.60 mmol, 3.0 equiv. ), 1,3-diene 4 (0.20 mmol), MeCN (0.5 mL), NEt 3 (56 μL) at room temperature. The reaction tube was sealed with a Teflon screw cap, removed from the glove box. Then, the reaction mixture was stirred at 80 °C for 24 h. The ratio of 5 and 5’ was determined by GC-FID analysis. And the crude reaction mixture was purified by column chromatography on silica gel or recrystallization using petroleum ether and dichloromethane to afford the corresponding product 5 . General procedure for Ni-catalyzed branched Heck reaction of 1,3-dienes In a glove box, Ni(cod) 2 (0.02 mmol, 10 mol%), IPr·HCl (0.024 mmol, 12 mol%), Cs 2 CO 3 (0.30 mmol, 1.5 equiv. ), and B1 /NaF (0.04 mmol, 20 mol%) were added to DMF (0.30 mL) in sequence and stirred at room temperature for 30 min. Then, the mixture of aryl triflate 1 (0.20 mmol), 1,3-diene 4 (0.30 mmol) in hexane (0.20 mL) was added into the reaction solvent. 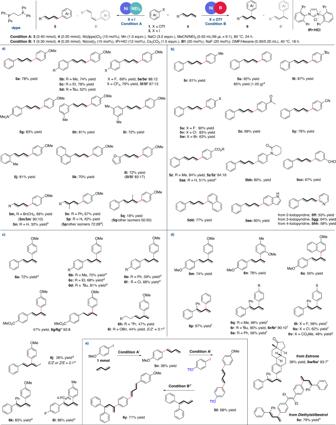Fig. 2: Substrate scope towards divergent Heck reactions. aSubstrate scopes of dienes for linear products.bSubstrate scopes of Ar-I for linear products.cSubstrate scopes of dienes for branched products.dSubstrate scopes of Ar-OTf for branched products.eCascade Heck reactions. Isolated yields were given in all cases. Selectivities were >20:1 except for some cases with footnotes, which were determined by GC-FID or1H NMR analysis.aiodobenzene (9.0 mmol),4a(6.0 mmol);b3a(0.20 mmol), 1,3-diene (0.60 mmol);cIsolated yield of two steps (coversion of -CO2H to -CO2Me);d1(0.20 mmol),4(0.25 mmol), 4-CNC6H4Bneop (B2, 20 mol%) was used instead ofB1;eA mixture ofZ- andE-isomers of diene4was used;f1(0.25 mmol);g1(0.20 mmol),4(0.25 mmol), KOtBu was used instead of NaF;h1(0.10 mmol),4(0.25 mmol), Ni(cod)2(20 mol%), IPr∙HCl (24 mol%), Cs2CO3(3.0 equiv.),B1(40 mol%), KOtBu (40 mol%);i3a(1.0 mmol), 1,3-butadiene (3.0 mmol), MeCN/NEt3(5.0 mL/0.60 mL = 9:1);jAr-I (0.60 mmol),5n(0.40 mmol), MeCN/NEt3(1.0 mL/0.11 mL = 9:1). The reaction tube was sealed with a Teflon screw cap, removed from the glove box. And the reaction mixture was stirred at 40 °C for 18 h. The selectivity was determined by 1 H NMR analysis. 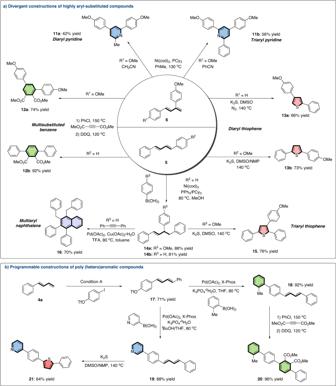Fig. 3: Divergent and programmable synthetic transformations of dienes. aDivergent constructions of highly aryl-substituted compounds.bProgrammable constructions of poly (hetero)aromatic compounds. 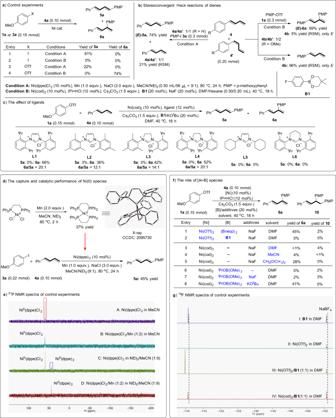Fig. 4: Mechanistic studies of Heck reactions. aControl experiments.bStereoconvergent Heck reactions of dienes.cThe effect of ligands.dThe capture and catalytic performance of Ni(0) species.e31P NMR spectra of control experiments.fThe role of [Ar-B] species.g19F NMR spectra of control experiments. 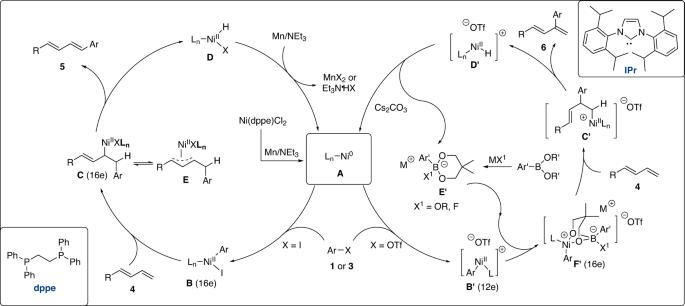Fig. 5: Proposed mechanism for divergent arylation via nickel catalysis. Through the regulation of dppe ligand, linear Heck product5is obtained in presence of Mn and NEt3. With the aid of bulky ligand IPr, the selectivity of reaction is switched to branched product6in presence of alkoxyborate. And the crude reaction mixture was purified by column chromatography on silica gel or recrystallization using petroleum ether and ethyl acetate to afford the corresponding product 6 .